Heparanase is a host enzyme required for herpes simplex virus-1 release from cells Herpesviruses exemplified by herpes simplex virus-1 (HSV-1) attach to cell surface heparan sulfate (HS) for entry into host cells. However, during a productive infection, the HS moieties on parent cells can trap newly exiting viral progenies and inhibit their release. Here we demonstrate that a HS-degrading enzyme of the host, heparanase (HPSE), is upregulated through NF-kB and translocated to the cell surface upon HSV-1 infection for the removal of HS to facilitate viral release. We also find a significant increase in HPSE release in vivo during infection of murine corneas and that knockdown of HPSE in vivo inhibits virus shedding. Overall, we propose that HPSE acts as a molecular switch for turning a virus-permissive ‘attachment mode’ of host cells to a virus-deterring ‘detachment mode’. Since many human viruses use HS as an attachment receptor, the HPSE-HS interplay may delineate a common mechanism for virus release. Herpesviruses cause one of the most prevalent human infections worldwide, with almost all eight viruses infecting a majority of the world population [1] . Among a number of other pathologies, HSV-1 is known to cause distressing infection of the human cornea, with HSV keratitis as the leading cause of infectious blindness in developed nations. Although acyclovir and its analogues are currently used for treatment of active herpes infections, these drugs fail to prevent permanent establishment of viral latency, allowing the virus to reactivate and cause clinical disease at a later time [2] . In order to generate more effective therapies, there is a critical need to understand the mechanism of viral spread to other cells and parts of the body after initial inoculation. The mechanism of HSV egress from cells largely remains a mystery; however, it is known that HSV-1 uses heparan sulfate (HS) as an attachment as well as an entry receptor for infection of host cells [1] , [3] . HS is an evolutionarily conserved glycosaminoglycan present ubiquitously at the cell surface and extracellular matrix of a wide range of cell types [4] . Viral glycoproteins gB, gC and gD are primarily responsible for viral binding to HS chains that are present on host cell surfaces as part of many proteoglycans including syndecans [1] , [5] , [6] . During viral egress, however, this important interaction has not been studied. Viral progenies have functional gB, gC and gD, and interactions of these glycoproteins with HS on parent cells during egress could significantly hamper their release. In this paper, we provide novel evidence that surface HS levels of infected cells are dramatically decreased by the infection-induced host enzyme heparanase-1 (HPSE). In normal cell physiology, HPSE plays a homeostatic role in regulating the turnover of cell-associated HS [7] . Here, we show that the upregulation of HPSE upon infection serves as a means for newly produced virions to avoid re-attachment to HS and re-entry into parent cells, thus increasing viral spread. Our evidence suggests that unlike influenza viruses, which encode neuraminidase for the removal of their attachment receptor during exit, herpesviruses are supported by a host enzyme for this key step in their life cycle. Loss of HS from the cell surface after infection During our quest to develop a new intervention against HSV infection, we attempted to use our newly discovered anti-HS peptides for preferentially targeting infected cells, and examined HS levels on the host cell surface [5] . We have previously shown that HS expression is increased during the initial stages of HSV-1 infection, and that this initial increase in HS expression enhances virus attachment to cells [6] . Quite unexpectedly, when we extended our study to longer time points, a dramatic decrease in HS was seen during later stages of infection (24 and 36 h). Both flow cytometry and immunofluorescence microscopy results demonstrated a continuous loss of HS from the surface of human corneal epithelial (HCE) cells, using HS antibody 10E4, US Biological ( Fig. 1a,b ). This phenomenon was also observed in HeLa cells ( Fig. 1c ). To examine the cause for decreased HS expression, an enzyme-linked immunosorbent assay (ELISA) kit was used to measure HS degradation after infection. At 24 and 36 h post infection (hpi), HS in infected cells was degraded at higher rates than in uninfected cells ( Fig. 1d ). This result implicated the only known mammalian HS-degrading enzyme, HPSE, in the loss of HS seen late during HSV-1 infection. 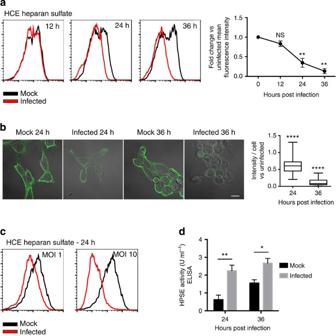Figure 1: Loss of HS from cell surface after infection. (a)Left—HS expression is decreased on the HCE cell surface at different time points post infection, measured using flow cytometry. Cells were infected with KOS-WT at MOI 0.1 and were stained for HS at 12, 24 and 36 hpi with HS antibody 10E4.Right—fluorescence intensity measurements based on flow cytometry results. Integrated mean fluorescence intensity of the whole population was measured and fold change was normalized to uninfected mock samples for each time point. (b)Left—representative immunofluorescence microscopy images show a decrease in HS expression on HCE cell surface of 24 and 36 hpi samples when compared with mock images. Cells were infected with KOS-WT at MOI 0.1 and were stained with HS antibody 10E4. Green represents HS expression. Images are merged with brightfield to show cell borders. Scale bar, 10 μm.Right—images were quantified for HS intensity. Eighty cells were picked at random from each sample and intensity of HS was measured for each cell using IMAGE J. (c) HS expression is decreased on HeLa cell surface after infection, measured using flow cytometry. Cells were infected with KOS-WT at MOIs of 1 and 10 for 24 h, and then stained for HS using HS antibody 10E4. (d) ELISA measurement of HPSE activity indicates increased degradation of HS upon infection. Infected cells showed more HS degradation activity when compared with uninfected cells at each time point. Increased HPSE activity was observed in uninfected cells at 36 h due to expansion of the number of cells in culture; the assay provides a measurement of the total amount of HPSE produced rather than on a per cell basis. All data are presented as mean±s.e.m. of three independent experiments (n=3). Asterisks denote a significant difference as determined by Student’st-test; *P<0.05, **P<0.01, ****P<0.0001. Figure 1: Loss of HS from cell surface after infection. ( a ) Left —HS expression is decreased on the HCE cell surface at different time points post infection, measured using flow cytometry. Cells were infected with KOS-WT at MOI 0.1 and were stained for HS at 12, 24 and 36 hpi with HS antibody 10E4. Right— fluorescence intensity measurements based on flow cytometry results. Integrated mean fluorescence intensity of the whole population was measured and fold change was normalized to uninfected mock samples for each time point. ( b ) Left— representative immunofluorescence microscopy images show a decrease in HS expression on HCE cell surface of 24 and 36 hpi samples when compared with mock images. Cells were infected with KOS-WT at MOI 0.1 and were stained with HS antibody 10E4. Green represents HS expression. Images are merged with brightfield to show cell borders. Scale bar, 10 μm. Right— images were quantified for HS intensity. Eighty cells were picked at random from each sample and intensity of HS was measured for each cell using IMAGE J. ( c ) HS expression is decreased on HeLa cell surface after infection, measured using flow cytometry. Cells were infected with KOS-WT at MOIs of 1 and 10 for 24 h, and then stained for HS using HS antibody 10E4. ( d ) ELISA measurement of HPSE activity indicates increased degradation of HS upon infection. Infected cells showed more HS degradation activity when compared with uninfected cells at each time point. Increased HPSE activity was observed in uninfected cells at 36 h due to expansion of the number of cells in culture; the assay provides a measurement of the total amount of HPSE produced rather than on a per cell basis. All data are presented as mean±s.e.m. of three independent experiments ( n =3). Asterisks denote a significant difference as determined by Student’s t- test; * P <0.05, ** P <0.01, **** P <0.0001. Full size image HPSE is upregulated after HSV-1 infection Since HS loss was increased after infection, we investigated HPSE expression in infected cells. Western blot analysis revealed that expression of active HPSE (50 kDa) was significantly greater at 24 and 36 hpi than in uninfected cells ( Fig. 2a ). Quantitative PCR (qPCR) revealed that HPSE mRNA was significantly elevated at 24 and 36 hpi ( Fig. 2b ). Furthermore, when HCE cells were transfected with HPSE promoter fused to luciferase reporter, an increase in luciferase expression was observed at 12, 24 and 36 hpi, when compared with uninfected mock-treated cells ( Fig. 2c ). We thus concluded that HPSE expression is regulated at the transcriptional level, with an increase in active HPSE protein produced upon HSV-1 infection. Interestingly, we observed similar increases in HPSE transcript levels ( Fig. 2d ) and protein expression levels ( Supplementary Fig. 1a ) after infection of HCE cells with other herpesviruses, namely herpes simplex virus type-2 (HSV-2), cytomegalovirus (CMV), bovine herpes virus and pseudorabies virus. In addition, an increase in HPSE was observed in various cell types when infected with HSV-1 KOS-WT ( Supplementary Fig. 1b ). HPSE upregulation seems to be a phenomenon common to multiple herpes viral infections and various cell types. As HPSE expression is increased inside the cells, we asked whether HPSE is translocated to the surface, the primary location of its substrate HS. Complementary to our HS expression results, a significant increase in HPSE was observed using flow cytometry and immunofluorescence microscopy at 24 and 36 hpi ( Fig. 2e,f ). It is known that both active HPSE (50 kDa) and inactive HPSE (65 kDa) can be found on the cell surface [7] . By isolating cell surface proteins and probing for HPSE by western blot analysis, we observed that only active 50-kDa HPSE is present at the cell surface at 24 and 36 hpi ( Supplementary Fig. 2a ). See Supplementary Fig. 9 for full-length images of supplementary figure gels and blots. Together, these results suggest that infected cells upregulate active HPSE, which is then translocated to the cell surface, producing the decreased HS expression observed on the cell surface after infection. 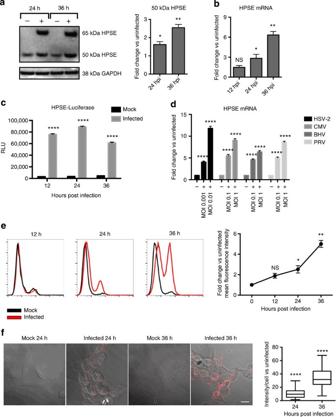Figure 2: HPSE is upregulated after HSV-1 infection. (a)Left—western blot shows increased expression of latent (65 kDa) and active (50 kDa) HPSE after 24 and 36 h infection of HCE cells at MOI 0.1.Right—densitometry quantification of 50 kDa active HPSE normalized to GAPDH. Fold change of infected over uninfected cells is shown for each time point. (b) Increase in HPSE transcripts in HCE cells after infection with KOS-WT at MOI 0.1. Results are shown as fold change of infected over uninfected cells at each time point, normalized to GAPDH. (c) Increase in promoter activity of theHPSEgene upon infection in HCE cells. KOS-WT was used to infect cells at MOI 0.1 for 12, 24 and 36 h. Shown is the average fold increase over uninfected control. Experimental values are normalized to those obtained with pGL3 as a control for transfection efficiency. (d) Increase in HPSE transcripts when cells were infected with HSV-2, CMV, bovine herpes virus (BHV) and pseudorabies virus (PRV). HCE cells were used for HSV-2, BHV and PRV infections, whereas primary human foreskin fibroblasts (HFF) were used for CMV infections. HCE cells were infected for 24 h. HFFs were infected with CMV for 7 days at indicated MOIs. Results are shown as fold change of infected over uninfected cells at each time point, normalized to GAPDH. (e)Left—HPSE expression is increased on cell surface after infection, measured using flow cytometry. HCE cells were infected with KOS-WT at MOI 0.1 and were stained with HPSE antibody HP130.Right—the integrated mean fluorescence intensity of the whole population was measured and fold change was normalized to mock at each time point. (f)Left—immunofluorescence microscopy images show increased HPSE expression on surface of infected HCE cells. Red represents HPSE expression. Images are merged with brightfield to show cell borders. Scale bar, 10 μm.Right—images were quantified for HPSE intensity. Eighty cells were picked at random for each sample and intensity of HPSE was measured for each cell using IMAGE J. All data are presented as mean±s.e.m. of three independent experiments (n=3). Asterisks denote a significant difference as determined by Student’st-test; *P<0.05, **P<0.01, ****P<0.0001, ns, not significant. SeeSupplementary Fig. 8for full-length images of blots. Figure 2: HPSE is upregulated after HSV-1 infection. ( a ) Left —western blot shows increased expression of latent (65 kDa) and active (50 kDa) HPSE after 24 and 36 h infection of HCE cells at MOI 0.1. Right —densitometry quantification of 50 kDa active HPSE normalized to GAPDH. Fold change of infected over uninfected cells is shown for each time point. ( b ) Increase in HPSE transcripts in HCE cells after infection with KOS-WT at MOI 0.1. Results are shown as fold change of infected over uninfected cells at each time point, normalized to GAPDH. ( c ) Increase in promoter activity of the HPSE gene upon infection in HCE cells. KOS-WT was used to infect cells at MOI 0.1 for 12, 24 and 36 h. Shown is the average fold increase over uninfected control. Experimental values are normalized to those obtained with pGL3 as a control for transfection efficiency. ( d ) Increase in HPSE transcripts when cells were infected with HSV-2, CMV, bovine herpes virus (BHV) and pseudorabies virus (PRV). HCE cells were used for HSV-2, BHV and PRV infections, whereas primary human foreskin fibroblasts (HFF) were used for CMV infections. HCE cells were infected for 24 h. HFFs were infected with CMV for 7 days at indicated MOIs. Results are shown as fold change of infected over uninfected cells at each time point, normalized to GAPDH. ( e ) Left— HPSE expression is increased on cell surface after infection, measured using flow cytometry. HCE cells were infected with KOS-WT at MOI 0.1 and were stained with HPSE antibody HP130. Right— the integrated mean fluorescence intensity of the whole population was measured and fold change was normalized to mock at each time point. ( f ) Left— immunofluorescence microscopy images show increased HPSE expression on surface of infected HCE cells. Red represents HPSE expression. Images are merged with brightfield to show cell borders. Scale bar, 10 μm. Right— images were quantified for HPSE intensity. Eighty cells were picked at random for each sample and intensity of HPSE was measured for each cell using IMAGE J. All data are presented as mean±s.e.m. of three independent experiments ( n =3). Asterisks denote a significant difference as determined by Student’s t- test; * P <0.05, ** P <0.01, **** P <0.0001, ns, not significant. See Supplementary Fig. 8 for full-length images of blots. Full size image Mechanism of HPSE upregulation upon infection In our search for the mechanism of HPSE upregulation upon infection, we learned from prior studies that a host factor, nuclear factor (NF)-kB, can transcriptionally increase HPSE expression [8] , [9] , [10] , [11] . A number of reports have also described an increased expression of the transcription factor NF-kB after HSV-1 infection [12] , [13] , [14] , [15] . Therefore, while studying a possible connection between NF-kB and HPSE upregulation during HSV-1 infection, we also observed a steady increase in NF-kB p65 levels ( Fig. 3a ), and increased nuclear translocation of the p65 subunit at 24 and 36 hpi ( Fig. 3b,c ). Thus, on the basis of previous reports [8] , [9] , [10] , [11] and our observations, it is likely that NF-kB activation during infection plays a role in HPSE induction. Adding support to this possibility, a similar phenomenon was reproduced when uninfected HCE cells were treated with an NF-kB inducer, Betulinic acid [16] . Quite evidently, NF-kB nuclear translocation and, more importantly, HPSE mRNA upregulation were observed ( Fig. 3d ). The role of NF-kB was further evaluated by overexpressing a plasmid encoding mutant IkBa (S32A/S36A) in HCE cells. This dominant-negative mutant is incapable of being phosphorylated and degraded [17] . Clearly, expression of the IkBa mutant inhibited NF-kB activation and its translocation to the nucleus, and we noted a decrease in HPSE expression by luciferase assay and qPCR ( Fig. 3e,f ). Collectively, our results indicate that NF-kB or one of its downstream effectors is directly involved in regulation of HPSE expression. In parallel studies, to probe any direct involvement of viral proteins in HPSE upregulation, we examined several known transcriptional regulators encoded in the HSV genome. HCE cells were separately transfected with expression plasmids for ICP0, ICP4, ICP22 and VP16, incubated for 24 h, and harvested for RNA isolation. No significant change in HPSE expression was observed using qPCR ( Supplementary Fig. 3a ). Together, these findings suggest that the upregulation of HPSE is likely a host response to infection that the virus takes advantage of to enhance its release from the parent cell. 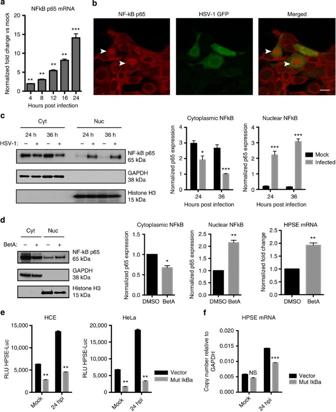Figure 3: Mechanism of HPSE upregulation upon infection. (a) Increase in NF-kB p65 transcript levels after infection with KOS-WT at MOI 0.1 at various time points. Results are normalized to GAPDH and reported as fold change of infected over uninfected cells. (b) Nuclear translocation of NF-kB p65 upon HSV-1 infection, observed using immunofluorescence microscopy. HCE cells were infected with GFP-KOS at MOI 0.1 for 24 h. Translocation of NF-kB to the nucleus can be seen in GFP-positive cells (arrowheads). Scale bar, 10 μm. (c) Nuclear translocation of NF-kB p65 upon HSV-1 infection measured by western blot analysis shows an increase in NF-kB translocation from the cytoplasm to the nucleus.Left—HCE cells were infected with KOS-WT at MOI 0.1 for 24 and 36 h, and nuclear/cytoplasmic extractions were performed.Right—densitometry quantification of NF-kB p65 in the cytoplasm and nucleus, normalized to GAPDH and Histone H3, respectively. (d) Induction of NF-kB activation by Betulinic acid (BetA) increases HPSE mRNA.Left—HCE cells were treated with BetA at 10 μg ml−1or DMSO vehicle for 24 h. NF-kB translocation into the nucleus with the BetA treatment is shown in HCE cells. Moreover, shown is densitometry quantification of NF-kB p65 in the cytoplasm and nucleus, normalized to GAPDH and Histone H3, respectively.Right—HPSE mRNA is increased with BetA treatment of HCE cells. (e) Inhibition of NF-kB activation results in decreased HPSE promoter activity. HCE cells (left) and HeLa cells (right) were transfected with mutant IkBa incapable of degradation (S32A/S36A), thereby specifically inhibiting NF-kB activation and nuclear translocation. Cells were infected with KOS-WT at MOI 0.1 for 24 h. Cell lysates were isolated, and luciferase assay was performed. Results shown are normalized to empty pGL3 vector as a control for transfection efficiency. (f) Inhibition of NF-kB activation results in decreased HPSE transcript levels upon infection. HCE cells were transfected with mutant IkBa as described above, and infected with KOS-WT at MOI 0.1 for 24 h. All data are presented as mean±s.e.m. of three independent experiments (n=3). Asterisks denote a significant difference as determined by Student’st-test; *P<0.05, **P<0.01, ***P<0.001, ****P<0.0001, ns, not significant. SeeSupplementary Fig. 8for full-length images of blots. Figure 3: Mechanism of HPSE upregulation upon infection. ( a ) Increase in NF-kB p65 transcript levels after infection with KOS-WT at MOI 0.1 at various time points. Results are normalized to GAPDH and reported as fold change of infected over uninfected cells. ( b ) Nuclear translocation of NF-kB p65 upon HSV-1 infection, observed using immunofluorescence microscopy. HCE cells were infected with GFP-KOS at MOI 0.1 for 24 h. Translocation of NF-kB to the nucleus can be seen in GFP-positive cells (arrowheads). Scale bar, 10 μm. ( c ) Nuclear translocation of NF-kB p65 upon HSV-1 infection measured by western blot analysis shows an increase in NF-kB translocation from the cytoplasm to the nucleus. Left— HCE cells were infected with KOS-WT at MOI 0.1 for 24 and 36 h, and nuclear/cytoplasmic extractions were performed. Right— densitometry quantification of NF-kB p65 in the cytoplasm and nucleus, normalized to GAPDH and Histone H3, respectively. ( d ) Induction of NF-kB activation by Betulinic acid (BetA) increases HPSE mRNA. Left— HCE cells were treated with BetA at 10 μg ml −1 or DMSO vehicle for 24 h. NF-kB translocation into the nucleus with the BetA treatment is shown in HCE cells. Moreover, shown is densitometry quantification of NF-kB p65 in the cytoplasm and nucleus, normalized to GAPDH and Histone H3, respectively. Right —HPSE mRNA is increased with BetA treatment of HCE cells. ( e ) Inhibition of NF-kB activation results in decreased HPSE promoter activity. HCE cells (left) and HeLa cells (right) were transfected with mutant IkBa incapable of degradation (S32A/S36A), thereby specifically inhibiting NF-kB activation and nuclear translocation. Cells were infected with KOS-WT at MOI 0.1 for 24 h. Cell lysates were isolated, and luciferase assay was performed. Results shown are normalized to empty pGL3 vector as a control for transfection efficiency. ( f ) Inhibition of NF-kB activation results in decreased HPSE transcript levels upon infection. HCE cells were transfected with mutant IkBa as described above, and infected with KOS-WT at MOI 0.1 for 24 h. All data are presented as mean±s.e.m. of three independent experiments ( n =3). Asterisks denote a significant difference as determined by Student’s t- test; * P <0.05, ** P <0.01, *** P <0.001, **** P <0.0001, ns, not significant. See Supplementary Fig. 8 for full-length images of blots. Full size image Functional phenotype of HPSE on viral egress and attachment To elucidate the role of higher HPSE production and associated enzymatic activity in viral egress, we transfected HCE cells with a HPSE expression plasmid and quantified the virus particles released in the cell culture supernatants at different time points by a plaque assay and viral DNA PCR. It was evident that viral release was increased in HPSE-transfected cells at 24, 36 and 48 hpi ( Fig. 4a ). To verify that the DNA PCR assay is suitable to detect the viral titre, a standard curve was calculated ( Supplementary Fig. 4a ). Conversely, using the same assays, we observed a loss of virus in the supernatant when HPSE was knocked down using lentiviral short hairpin RNA (shRNA) constructs ( Fig. 4b ). Loss of HPSE expression in knockdown cells is shown in Supplementary Fig. 5a . Furthermore, in support of a direct role in egress, we found that active, functional HPSE is required for efficient viral egress, as transfection of various nonfunctional HPSE mutants produced a defect in viral release ( Supplementary Fig. 6a ). According to our proposed mechanism, active HPSE is overexpressed inside cells and is translocated to the cell surface during viral egress to cleave HS, which facilitates increased viral shedding from cells. To prove that higher HPSE expression is the cause of HS loss at the surface, we transfected HCE cells with HPSE plasmid in the absence of any infection and found that HS levels start to decrease at 24 h post transfection ( Fig. 4c ). To delve deeper into the role of HPSE activity in viral release, we performed a viral attachment assay, which confirmed that a loss in HS decreases viral binding at the surface ( Fig. 4d ). Next, to further understand HSV egress under physiological conditions, we tested binding of exogenous GFP (green fluorescent protein) HSV-1 to cells that had already been infected with wild-type virus. We hypothesized that if HS levels decrease during the later stages of infection, any exogenous virions added to already infected cells should demonstrate a loss of binding to the surface. Indeed, compared with uninfected cells, the binding of exogenous GFP virus to the surface of wild-type virus-infected cells (24 and 36 hpi) was decreased ( Fig. 4e ). Together, these results suggest that HSV-1-infected cells become less prone to virus attachment as they start to release their progeny virions. Given our findings of an inverse relationship between HS and HPSE expression, we propose that HPSE is a switch needed to convert the cell from a virus-permissive ‘attachment mode’ to a virus-deterring ‘detachment mode’ during the productive period of infection ( Fig. 4f ). 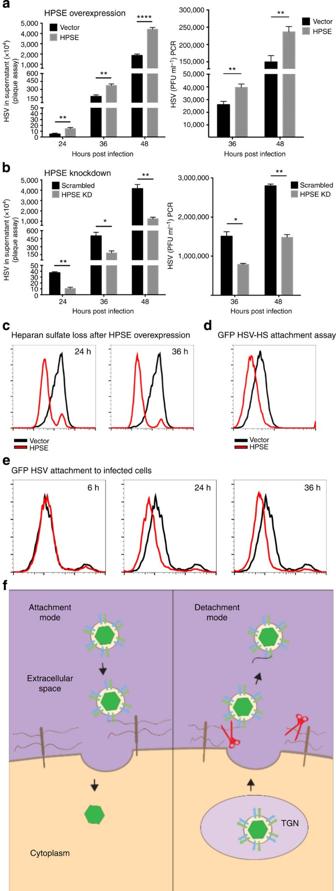Figure 4: Functional phenotype of HPSE on viral egress and attachment. (a) Viral egress is increased in HPSE-overexpressing cells.Left—HCE cells were infected with KOS-WT at MOI 0.1 24 h after transfection with HPSE or control vector. Supernatant was collected at indicated time points post infection and virus was quantified by titering on Vero cells in a plaque assay.Right—HCE cells were transfected and infected as mentioned above and culture supernatant containing viruses were collected and quantified with PCR using primers against glycoprotein-D (gD). (b) Viral egress is decreased in HPSE-deficient cells. Stably transduced HCE cell lines were generated using lentiviral HPSE shRNA and scrambled shRNA constructs, and these were then infected with KOS-WT at MOI 0.1. As described above, the supernatant was collected to perform plaque assay (left) and viral DNA was quantified using PCR for gD (right). (c) HS is lost from the cell surface on HPSE overexpression. HCE cells were transfected with HPSE plasmid or control vector, incubated at 37 °C for 24 h. Cells were then stained for HS using antibody 10E4 at 24 and 36 hpi and analysed with flow cytometry. (d) Decreased attachment of HSV-1 after HPSE overexpression. HCE cells were transfected with HPSE plasmid or control vector, and 24 h later incubated with GFP-KOS for 2 h at 4 °C to allow viral binding. GFP fluorescence intensity from the virus was measured using flow cytometry. (e) Decreased attachment of GFP-KOS after previous infection with KOS-WT at specified time points. HCE cells were infected with KOS-WT for 6, 24 or 36 h, and then incubated with GFP-KOS for 2 h at 4 °C to allow viral binding. GFP fluorescence intensity from the virus was measured using flow cytometry. Black curve represents 0-h time point. (f) Model of HSV egress, showing the role of HPSE at the cell surface. This model shows the attachment and detachment modes of the HSV lifecycle. During attachment, virus is bound to HS. However, during detachment HPSE (red) is upregulated and translocated to the cell surface, cleaving HS to allow viral exit. All data are presented as mean±s.e.m. of three independent experiments (n=3). Asterisks denote a significant difference as determined by Student’st-test; *P<0.05, **P<0.01, ****P<0.0001. Figure 4: Functional phenotype of HPSE on viral egress and attachment. ( a ) Viral egress is increased in HPSE-overexpressing cells. Left— HCE cells were infected with KOS-WT at MOI 0.1 24 h after transfection with HPSE or control vector. Supernatant was collected at indicated time points post infection and virus was quantified by titering on Vero cells in a plaque assay. Right —HCE cells were transfected and infected as mentioned above and culture supernatant containing viruses were collected and quantified with PCR using primers against glycoprotein-D (gD). ( b ) Viral egress is decreased in HPSE-deficient cells. Stably transduced HCE cell lines were generated using lentiviral HPSE shRNA and scrambled shRNA constructs, and these were then infected with KOS-WT at MOI 0.1. As described above, the supernatant was collected to perform plaque assay (left) and viral DNA was quantified using PCR for gD (right). ( c ) HS is lost from the cell surface on HPSE overexpression. HCE cells were transfected with HPSE plasmid or control vector, incubated at 37 °C for 24 h. Cells were then stained for HS using antibody 10E4 at 24 and 36 hpi and analysed with flow cytometry. ( d ) Decreased attachment of HSV-1 after HPSE overexpression. HCE cells were transfected with HPSE plasmid or control vector, and 24 h later incubated with GFP-KOS for 2 h at 4 °C to allow viral binding. GFP fluorescence intensity from the virus was measured using flow cytometry. ( e ) Decreased attachment of GFP-KOS after previous infection with KOS-WT at specified time points. HCE cells were infected with KOS-WT for 6, 24 or 36 h, and then incubated with GFP-KOS for 2 h at 4 °C to allow viral binding. GFP fluorescence intensity from the virus was measured using flow cytometry. Black curve represents 0-h time point. ( f ) Model of HSV egress, showing the role of HPSE at the cell surface. This model shows the attachment and detachment modes of the HSV lifecycle. During attachment, virus is bound to HS. However, during detachment HPSE (red) is upregulated and translocated to the cell surface, cleaving HS to allow viral exit. All data are presented as mean±s.e.m. of three independent experiments ( n =3). Asterisks denote a significant difference as determined by Student’s t- test; * P <0.05, ** P <0.01, **** P <0.0001. Full size image Significance of HPSE and HSV egress in vivo Mouse corneas were injected with vectors containing shRNA against murine HPSE or scrambled sequence, and then infected with GFP HSV. Decreased viral spread through the cornea was observed with HPSE knockdown ( Fig. 5a ). Swabs collected from knockdown corneas at 24 and 72 hpi produced fewer plaques when compared with eyes with scrambled shRNA ( Fig. 5b , left). This suggests that HPSE activity promotes viral egress in the epithelium of the cornea. Furthermore, using fluorescein dye we detected decreased tissue damage in HPSE knockdown corneas infected with wild-type virus, as compared with corneas of mice that received scrambled sequence ( Fig. 5b , right). Conversely, when mouse eyes were transfected with HPSE and then infected with HSV-1, more virus was present as measured by corneal swabs ( Fig. 5c , left). In addition, these HPSE-overexpressing corneas displayed increased corneal ulceration and tissue damage when compared with empty vector transfected corneas ( Fig. 5c , right). To further establish HPSE’s significance in disease, the four aforementioned groups of mice were observed using slit lamp biomicroscope 7 days post-ocular infection and assigned clinical scores according to pre-established criteria [18] . HPSE knockdown produced fewer signs of keratitis, while HPSE overexpression resulted in exaggerated disease ( Fig. 5d ). In addition, treating mice with heparin, a HPSE inhibitor, resulted in less virus being present in the corneal swabs ( Fig. 5e ). Together, these results indicate that HPSE activity promotes viral egress in the corneal epithelium, contributing to the tissue damage characteristic of herpetic keratitis. Last, we aimed to determine whether HSV could upregulate HPSE expression in human tissue. Epithelial cells of human donor corneoscleral buttons infected with HSV showed increased levels of active HPSE ( Fig. 5f ). This suggests that the virus–HPSE association is relevant in human pathogenesis as well. 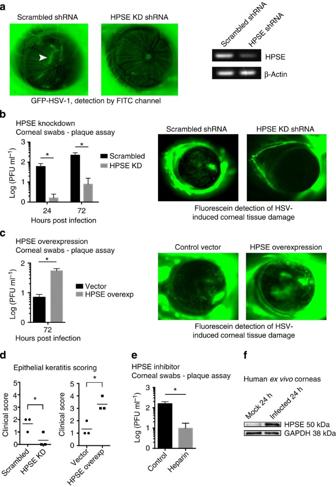Figure 5: Significance of HPSE and HSV egressin vivo. (a) Knockdown of HPSE in mouse eyes decreases viral spread through the cornea. Mouse corneas were injected with shRNA against HPSE or with scrambled shRNA and infected with GFP-KOS.Left—fluorescence detection 72 h post infection. Arrowhead indicates GFP-HSV.Right—knockdown of HPSE in mouse cornea demonstrated by reverse transcriptase PCR. (b)Left—corneal eye swabs collected at 24 and 72 hpi for plaque assays show decreased HSV titre in HPSE knockdown corneas (n=5 for each group).Right—decreased corneal tissue damage in HPSE knockdown mouse corneas after HSV-1 infection. HPSE was knocked down in mouse corneas as described above, and 7 days post infection with KOS-WT, fluorescein was applied to mouse eyes to highlight corneal damage. (c)Left—mouse corneas were transfected with HPSE plasmid in the corneal epithelium and infected with KOS-WT. Corneal swabs collected at 72 hpi for plaque assays show an increase in HSV titre in the cornea transfected with HPSE plasmid (n=3 for each group).Right—increased corneal tissue damage in HPSE-overexpressing mouse corneas after HSV-1 infection. Fluorescein was applied to mouse eyes to highlight tissue damage 7 days post infection. (d) 7 days post ocular infection, mouse corneas were examined for tissue damage using slit lamp biomicroscope and scored.Left—decreased tissue damage in HPSE shRNA knockdown corneas when compared with scrambled shRNA controls.Right—increased tissue damage in HPSE-overexpressed corneas when compared with vector-transfected controls (n=3 for each group). (e) Decreased viral egress after heparin treatment, measured using the plaque assay. Mouse corneas were infected with KOS-WT at 105p.f.u. After infection, 5 μl of 25 μg μl−1heparin solution was applied directly to corneas at 24 and 48 hpi, and corneal swabs for plaque assay were collected at 72 hpi. (f) Human corneoscleral buttons from the same subject were cultured and infected with KOS-WT at 105p.f.u. The epithelium was extracted at 24 hpi and an increase in HSPE (50 kDa) was observed. The experiment was repeated three times and representative western blot analysis is shown. All data are presented as mean±s.e.m. of three independent experiments (n=3). Asterisks denote a significant difference as determined by Student’st-test; *P<0.05. SeeSupplementary Fig. 8for full-length images of gels and blots. Figure 5: Significance of HPSE and HSV egress in vivo. ( a ) Knockdown of HPSE in mouse eyes decreases viral spread through the cornea. Mouse corneas were injected with shRNA against HPSE or with scrambled shRNA and infected with GFP-KOS. Left —fluorescence detection 72 h post infection. Arrowhead indicates GFP-HSV. Right —knockdown of HPSE in mouse cornea demonstrated by reverse transcriptase PCR. ( b ) Left —corneal eye swabs collected at 24 and 72 hpi for plaque assays show decreased HSV titre in HPSE knockdown corneas ( n =5 for each group). Right —decreased corneal tissue damage in HPSE knockdown mouse corneas after HSV-1 infection. HPSE was knocked down in mouse corneas as described above, and 7 days post infection with KOS-WT, fluorescein was applied to mouse eyes to highlight corneal damage. ( c ) Left —mouse corneas were transfected with HPSE plasmid in the corneal epithelium and infected with KOS-WT. Corneal swabs collected at 72 hpi for plaque assays show an increase in HSV titre in the cornea transfected with HPSE plasmid ( n =3 for each group). Right —increased corneal tissue damage in HPSE-overexpressing mouse corneas after HSV-1 infection. Fluorescein was applied to mouse eyes to highlight tissue damage 7 days post infection. ( d ) 7 days post ocular infection, mouse corneas were examined for tissue damage using slit lamp biomicroscope and scored. Left —decreased tissue damage in HPSE shRNA knockdown corneas when compared with scrambled shRNA controls. Right —increased tissue damage in HPSE-overexpressed corneas when compared with vector-transfected controls ( n =3 for each group). ( e ) Decreased viral egress after heparin treatment, measured using the plaque assay. Mouse corneas were infected with KOS-WT at 10 5 p.f.u. After infection, 5 μl of 25 μg μl −1 heparin solution was applied directly to corneas at 24 and 48 hpi, and corneal swabs for plaque assay were collected at 72 hpi. ( f ) Human corneoscleral buttons from the same subject were cultured and infected with KOS-WT at 10 5 p.f.u. The epithelium was extracted at 24 hpi and an increase in HSPE (50 kDa) was observed. The experiment was repeated three times and representative western blot analysis is shown. All data are presented as mean±s.e.m. of three independent experiments ( n =3). Asterisks denote a significant difference as determined by Student’s t- test; * P <0.05. See Supplementary Fig. 8 for full-length images of gels and blots. Full size image HS is a ubiquitously expressed glycosaminoglycan that is used as a docking site by HSV-1. Glycoproteins gB, gC and gD mediate this initial contact of virus with host cell HS, which is followed by fusion, entry and eventually production of viral progeny [1] . These newly formed viral progenies have functional glycoproteins that could interact with HS during egress. Influenza virus also faces a similar predicament in which viral haemagglutinin binds to host sialic acid chains during egress. To avoid being trapped by parent host cells, these chains are cleaved with the help of the enzyme neuraminidase, which is encoded in the genome of the influenza virus [19] . In contrast, HSV-1 is not known to encode any enzymes in its genome that cleave HS chains. Hence, HSV and other herpesviruses could have found support from a host-derived enzyme, namely HPSE, to perform the task of cleaving HS chains. In addition to the cleavage of HS during infection, it is possible that entire proteoglycans are also being shed. It has been described previously that increased HPSE activity results in an increased rate of syndecan-1 shedding on the cell surface [20] . In this study, using slot blot of cell culture supernatants, we have observed a moderate increase in syndecan-1 shedding after HSV-1 infection ( Supplementary Fig. 7a ). Although the exact mechanism is not known, shedding of syndecan-1 because of HPSE could be attributable to HPSE-induced upregulation of host cell proteases such as MMP-9 (ref. 21 ). In this way, HPSE could play a dual role in viral egress by cleaving HS and the proteoglycan to which it is attached. However, we believe that the HPSE–HS association plays the major role in viral egress because viral dispersion is limited when bound to an entire proteoglycan rather than small HS chains. In addition, any shedding of syndecan proteoglycans probably plays a relatively minor role during viral egress since the bulky proteoglycan core would likely need to be removed before progeny entry into neighbouring cells. Another proteoglycan that plays a minor role in viral entry is chondroitin sulfate (CSPG) [22] . However, since the vast majority of literature shows that HSPGs are the primary receptors when compared with CSPGs, our current study is focused on the former. Future studies will aim to elucidate the mechanism of egress in relation to CSPGs. With the new evidence from this study, we propose two distinct modes in the life of infected cells, viral attachment and detachment modes, which are regulated by the host enzyme HPSE ( Fig. 4f ). During the attachment mode, HSV glycoproteins bind to HS at the cell surface, an interaction that facilitates viral entry. With the upregulation of HPSE upon infection, which coincides well with viral maturation and egress phases, the host cell transforms into the detachment mode by translocating HPSE to the plasma membrane, removing HS from the surface, and aiding in viral exit. Quite notably, HPSE is found to have four to five times increased enzymatic activity in an acidic environment of pH 6.4 when compared with pH 7.2 (ref. 23 ). Interestingly, the trans -Golgi network (TGN) also has a low pH value of 5.91 (ref. 24 ). Hence, when the TGN or TGN-derived vesicles fuse with the plasma membrane, it creates an acidic microenvironment promoting activation of HPSE, which in the case of infected cells can specifically increase the effectiveness of viral egress. All such events discussed above allow HPSE to act efficiently as a switch in infected cells, making them less prone to secondary infection by aggressive HS cleavage. Herpes viral glycoproteins use other cell surface receptors for entry, the most common of which being nectin-1. However, it has been shown that expression of nectin-1 is diminished before cell death in neuronal cells of infected mice and HCE cells during egress [25] , [26] . It is likely, although not well studied, that the surface expression of other HSV entry receptors is also diminished with infection. A more significant problem, therefore, is likely posed by the presence of HS on cell surfaces. Given the high abundance on cell surfaces and presence of highly charged groups, HS proteoglycans are considered most important for virus attachment to cells [1] , and are hence most likely to trap egressing virions. Adding further complexity, a single HS chain can bind multiple viral ligands. As an example, HS chains on human HEp-2 cells are on average 105 kDa in apparent molecular mass, which corresponds to 420 sugar residues per chain or a chain length of 190 nm. Thousands of such chains may be present on the surface of single cells. Hence, for the entire length of the proteoglycan, there exist multiple chances for it to be trapped by HS on the same cell [1] , [26] . Therefore, removal of HS moieties is likely to clear a big hurdle in viral release. HS proteoglycans are ubiquitously expressed glycosaminoglycans and are used by many viruses such as adeno-associated viruses [27] , dengue viruses [28] , hepatitis-C virus [29] , foot-and-mouth disease virus [30] , vaccinia virus [31] , yellow fever virus [32] , sindbis virus [33] , HIV [34] , papilloma virus [35] , cytomegalovirus [36] , human respiratory syncytial virus [37] and virtually all herpesviruses [1] for initial attachment to cells [27] , [28] , [29] , [30] , [31] , [32] , [33] , [34] , [35] , [36] , [37] , [38] . It is thus reasonable to assume that HPSE activity could play a role in the pathogenesis of these viruses as well. In fact, it has been reported that HPSE expression was significantly higher in Hepatitis C virus (HCV)-related hepatocellular carcinoma (HCC) patients when compared with HCV-negative HCC patient population [39] . It is likely that future studies will directly link HPSE activity to the release of virtually all viruses that rely on HS for attachment to their host cells. Interestingly, in an unrelated study, a potent HPSE inhibitor that is currently in human clinical trials for cancer treatment, PI-88, successfully decreased cell-to-cell spread of HSV-1 and HSV-2 (ref. 40 ). In ocular infection, distressing lesions caused by HSV-1 infection can result in vision impairment and blindness resulting from a chronic inflammatory reaction in the cornea causing neovascularization by limbal blood vessels [41] . Recent studies have implicated HPSE overexpression in multiple pathologic processes, including inflammation, angiogenesis, tumour metastasis and atherosclerosis [7] , [42] , [43] , [44] , [45] . By breaking down epithelial and endothelial basement membranes, HPSE produces increased vascular permeability and leukocyte extravasation [46] , and liberates HS-bound cytokines and growth factors normally sequestered in the extracellular matrix, making them available for angiogenesis and inflammation in the surrounding area [7] , [44] , [47] , [48] , [49] . Vision loss from HSV keratitis is predominantly due to corneal clouding caused by inflammation. In light of these recent findings, HPSE may be a unique therapeutic target since HPSE inhibitors could reduce viral release and control the host inflammatory response. Cells and viruses HCE cell line (RCB1834 HCE-T) was obtained from Kozaburo Hayashi (National Eye Institute, Bethesda, MD) and was cultured in MEM (Life Technologies, Carlsbad, CA) with 10% fetal bovine serum (FBS) and 1% penicillin/streptomycin. For convenience, this cell line is referred to as HCE cells throughout the paper. All infections were performed with HSV-1 KOS-WT at multiplicity of infection (MOI) of 0.1 on HCE cells unless mentioned otherwise. Primary human foreskin fibroblasts for CMV infections were provided by Dr Nell Lurain (Rush University, Chicago, IL). The African green monkey kidney (Vero), HEK293T, HeLa and mouse embryonic fibroblast cell lines were obtained from Dr Patricia G. Spear (Northwestern University, Chicago, IL) and cultured in DMEM (Life Technologies) with 10% FBS and 1% penicillin/streptomycin. Betulinic acid was purchased from R&D Systems (Minneapolis, MN) and was used at a concentration of 10 μg ml −1 in dimethylsulphoxide (DMSO) to induce NF-kB activation in cell cultures. The viruses used in this study, HSV-1 (KOS-WT) [50] , GFP-KOS [51] , pseudorabies virus [52] and bovine herpes virus [53] , were provided by Dr Patricia G. Spear (Northwestern University). CMV strain AD169 (ref. 54 ) was provided by Dr Nell Lurain (Rush University Medical Center, Chicago, IL). All virus stocks except for CMV were propagated in Vero cells and stored at −80 °C. CMV was propagated in human foreskin fibroblast cells. Antibodies and plasmids HPSE antibody HP130 (Advanced Targeting Systems, San Diego, CA) was used for western blot analysis (1:200), imaging (1:100) and flow cytometry studies (1:100). Histone H3 antibody (Cell Signaling Technology, Danvers, MA) was used at a dilution of 1:2,000 for western blot analysis. Anti-human HS monoclonal antibody 10E4 (US Biological, Salem, MA) was used for flow cytometry (1:50) and cell imaging (1:100). NF-kB p65 antibody C-20 (Santa Cruz Biotechnology) was used for imaging (1:500) and western blot analysis (1:2,000). GAPDH (Santa Cruz Biotechnology) was used for western blot analysis at dilution 1:2,000. Na + /K + -ATPase (Cell Signaling) was used for western blot analysis at dilution 1:20,000. Human HPSE expression plasmid pIRES2 EGFP-HPSE1 (HPSE) and the control empty vector pIRES2 EGFP plasmid [55] were provided by Dr Ralph Sanderson (University of Alabama at Birmingham, Birmingham, AL). Mutant IkBa (S32/36A) plasmid [17] was provided by Dr Michael Karin (University of California, San Diego, La Jolla, CA). Expression constructs for viral transcriptional regulators ICP0 (ref. 56 ) and VP16 were obtained from Dr Bernard Roizman (University of Chicago, Chicago, IL). VP16 plasmid was kindly prepared by Grace Zhou. VP16-coding sequence driven by the CMV promoter was inserted in MCS of pcDNA 3.1(+). The whole fragment was flanked by the VP16 gene flanking sequences for recombination purposes. The ICP4 plasmid [57] was obtained from Dr Neal DeLuca (University of Pittsburgh, Pittsburgh, PA). The ICP22 plasmid was kindly provided by Dr Kumar Penmetcha (National institute of Advanced Industrial Science and Technology, Ibaraki, Japan). ICP22-coding sequence driven by the CMV promoter was inserted in MCS of pcDNA 3.1(+). The whole fragment was flanked by ICP22 gene flanking sequences for recombination purposes. HPSE expression constructs GS-3, TIMB, C-domain and Delta 17 were a kind gift from Dr Israel Vlodavsky (Rappaport Institute, Haifa, Israel) [58] . All overexpression transfections were performed using Lipofectamine-2000 transfection reagent (Life Technologies), according to the manufacturer’s specifications. Western blot analysis Proteins from samples in this study were collected using radio immunoprecipitation assay (RIPA) buffer (Sigma-Aldrich, St Louis, MO) according to the manufacturer’s protocol. After gel electrophoresis, membranes were blocked in 5% milk/TBS-T for 1 h followed by incubation with primary antibody overnight. After washes and incubation with respective horseradish peroxidase-conjugated secondary antibodies (anti-mouse 1:10,000, anti-rabbit 1:20,000) for 1 h, protein bands were visualized using the SuperSignal West Femto maximum sensitivity substrate (Thermo Scientific, Waltham, MA) with ImageQuant LAS 4000 biomolecular imager (GE Healthcare Life Sciences, Pittsburgh, PA). The densities of the bands were quantified using the ImageQuant TL image analysis software (GE Healthcare Life Sciences). Supernatant slot blot Cell culture supernatants of infected or mock-treated HCE cells were vacuum-filtered through Immobilon-Ny+ nylon membrane (Millipore Corporation, Billerica, MA) using Bio-Dot SF apparatus (Bio-Rad, Hercules, CA). Membranes were blotted overnight with antibody specific for Syndecan-1 (Santa Cruz Biotechnology, sc-6532) followed by species-specific secondary antibody and chemiluminescence detection using ImageQuant LAS 4000 biomolecular imager (GE Healthcare Life Sciences), as described above. Nuclear protein extraction Cells were washed with cold PBS and collected using a cell scraper. Cells were then treated with hypotonic buffer (20 M Tris-HCl, pH 7.4, 10 mM NaCl, 3 mM MgCl 2 ) and 10% NP-40 and centrifuged. The pellet was treated with cell extraction buffer (Life Technologies) according to the company’s protocol to collect nuclear extract. Halt Protease and Phosphatase Inhibitor Cocktail (Thermo Scientific) was added to the samples and samples were stored in −80 °C until analysis. Cell surface protein extraction The Cell Surface Protein Isolation Kit (Thermo Scientific) was used to isolate proteins on the surface of the cell membrane. Briefly, cell surface proteins were labelled with sulfo-NHS-SS-Biotin and lysed. Biotinylated proteins from the remaining lysates were isolated using NeutrAvidin agarose columns, eluted and analysed with western blot analysis. PCR RNA was extracted from cells using Trizol (Life Technologies) according to the manufacturer’s protocol. RNA was then transcribed to DNA using High Capacity cDNA Reverse Transcription Kit (Applied Biosystems, Foster City, CA). Real-time quantitative PCR was performed using Fast SYBR Green Master Mix (Applied Biosystems) using QuantStudio 7 Flex (Applied Biosystems). The primers used in this study are as follows: HPSE forward primer 5′-CTCGAAGAAAGACGGCTA-3′ and reverse primer 5′-GTAGCAGTCCGTCCATTC-3′; viral glycoprotein gD forward primer 5′-TACAACCTGACCATCGCTTC-3′ and reverse primer 5′-GCCCCCAGAGACTTGTTGTA-3′; NF-kB p65 forward primer 5′-TGGGGACTACGACCTGAATG-3′ and reverse primer 5′-GGGGGCACGATTGTCAAAGA-3′; GAPDH forward primer 5′-TCCACTGGCGTCTTCACC-3′ and reverse primer 5′-GGCAGAGATGATGACCCTTTT-3′. Semi-quantitative RT–PCR was performed using the PCR Master Mix (Thermo Scientific) according to the manufacturer’s protocol. Human HPSE forward primer 5′-TTCGATCCCAAGAAGGAATCAAC-3′ and reverse primer 5′-GTAGTGATGCCATGTAACTGAATC-3′ for 25 cycles. Human GAPDH forward primer 5′-TCCACTGGCGTCTTCACC-3′ and reverse primer 5′-GGCAGAGATGATGACCCTTTT-3′ for 25 cycles. Mouse HPSE forward primer 5′-CAAGAACAGCACCTACTCAAG-3′ and reverse primer 5′-AGCAGTAGTCAAGGAGAAGC-3′ for 28 cycles. Mouse β-actin forward primer 5′-CGGTTCCGATGCCCTGAGGCTCTT and reverse primer 5′-CGTCACACTTCATGATGGAATTGA-3′ for 28 cycles. Luciferase assay pHep1(0.7 kb)-luc plasmid [59] expressing firefly luciferase driven by the 0.7-kb promoter area upstream of the transcription start site of human HPSE was provided by Dr Xiulong Xu (Rush University). Empty vector, pGL3-Basic (Promega, Madison, WI), was used as a control for transfection efficiency. Luciferase activity was measured using Berthold Luminometer. Flow cytometry HS and HPSE cell surface expression were detected after HSV-1 KOS-WT infection. Monolayers of HCE cells were infected at MOI 0.1 and harvested at different times post infection. The following procedure for detecting HS expression has been described previously [6] . Briefly, cells were harvested and incubated with primary antibody diluted in PBS with 1% BSA for 20 min at 4 °C followed by 30 min incubation with fluorescein isothiocyanate (FITC)-conjugated anti-mouse IgM diluted to 1:100. For detection of HPSE on the cell surface, cells were harvested and incubated with (3 μg per sample) primary antibody diluted in PBS with 1% BSA for 1 h at 4 °C and 30 min incubation with FITC-conjugated anti-mouse IgG diluted to 1:100. Cells stained with respective FITC-conjugated secondaries were used as background controls. Entire cell populations were used for the mean fluorescence intensity calculations. For GFP HSV attachment assay, cells were counted and incubated with GFP-KOS at MOI 1,000. Cells were allowed to adsorb the virus for 2 h at 4 °C in order to facilitate attachment to cell surface but prevent entry. Viral attachment with GFP-KOS virus was quantified using flow cytometry. Entire cell populations were used for the mean fluorescence intensity calculations. Flow cytometry was performed on a CyAn ADP Analyzer (Beckman Coulter, Brea, CA) and data were analysed using the FlowJo analysis software. Immunofluorescence microscopy HCE cells were cultured in glass bottom dishes (MatTek Corporation, Ashland, MA). Cells were fixed in 10% paraformaldehyde for 10 min and permeabilized with 0.1% Triton-X for 10 min for intracellular labelling. This was followed by incubation with primary antibody for 2 h at 4 °C. When a secondary antibody was needed, cells were incubated with FITC-conjugated secondary antibody at dilution 1:150 for 1 h and were examined under Zeiss Confocal 710, Germany using a × 63 oil objective lens. Pinhole was set to 1 Airy Unit. For cell surface staining, cells were incubated with respective antibodies before fixation with paraformaldehyde for imaging. Fluorescence intensity of images was calculated using Image J. Plaque assay Viral egress was measured using the plaque assay. Monolayers of HCE cells were plated in six-well plates and infected with KOS-WT virus at MOI 0.1. Media were collected at different time points post infection and titred on Vero cells. Briefly, primary incubation of collected media was performed with Opti-MEM (Life Technologies) for 2 h. Vero cells were then incubated with growth media containing 1% methylcellulose for 72 h followed by fixing with 100% methanol and staining with crystal violet solution. Virus titre using PCR Supernatant was collected from infected samples and viral DNA was purified using the QIAamp MinElute Virus Spin Kit (Qiagen, Venlo, the Netherlands). The extracted DNA was eluted in 20 μl and was subjected to qPCR (2 μl of DNA per sample) using HSV gD primers. To verify that this assay is suitable to detect changes in HSV, a standard curve was calculated ( Supplementary Fig. 4a ). A virus of known titre was serially diluted to five different dilutions, and the viral DNA was extracted to perform qPCR. The coefficient of determination ( R 2 ) of the standard curve was 0.999 and the equation calculated was used for determining the amount of virus present in the supernatant. HPSE activity ELISA HCE cells were infected with KOS-WT virus (MOI 0.1). At different times post infection, infected samples were used to measure HPSE activity using the Heparan Degrading Enzyme Assay Kit (Takara Bio Inc., Shiga, Japan). Briefly, infected samples were mixed 1:1 with reaction buffer and incubated for 45 min at 37 °C. This mix was transferred to wells coated with fibroblast growth factor, which binds undegraded HS, and incubated for 15 min at 37 °C, after which Avidin phenacetin O-de-ethylase conjugate was added and incubated for 45 min. Phenacetin O-de-ethylase substrate was added and absorbance at 450 nm was measured with a microplate reader. HPSE degradation activity (U ml −1 ) of samples was measured utilizing a standard curve. One unit is defined as the activity that can degrade 0.063 ng of biotinylated HS when reacted at pH 5.8 at 37 °C for 1 min. Mouse cornea nucleic acid delivery and ocular infection Animals were cared for and procedures were performed in accordance with the institutional and NIH guidelines and approved by the Animal Care Committee at the University of Illinois. Male and female Balb/c mice from Jackson Laboratory (Bar Harbor, ME) were used for animal experiments. Plasmids containing murine HPSE shRNA (Sigma-Aldrich, TRCN0000098111), scrambled shRNA, active HPSE GS-3 or empty vector were introduced into the epithelium using a previously established protocol [60] , [61] . Briefly, a nick in the epithelium and anterior stroma of mouse eyes were made with a 30-gauge needle. DNA (2 μl) was injected into the stroma using 33-gauge Hamilton syringe (Hamilton, Reno, NV). Fluorescence images of the eye were captured using a stereoscope (StereoLumar V.12, Carl Zeiss, GmbH, Hamburg, Germany) according to previously mentioned protocol [62] . Briefly, an anaesthetized mouse was placed on the stereoscope stage with mouse adaptor (RWD Lifesciences, San Diego, CA, Cat. No. 900-0068-010). Proparacaine (5 μl; 0.5%, Bausch & Lomb, Tampa, FL) was applied for 3 min, and the pupil was constricted with 5 μl 0.01% carbachol (Miostat Alcon, Fort Worth, TX) for 5 min before acquiring images. Mouse eyes were infected on Day 3 post transfection with KOS-WT virus or GFP-KOS (1 × 10 5 p.f.u. in 5 μl), according to the described protocol [63] . Swabs were collected on appropriate days according to the previously mentioned protocol [64] and plaque assay was performed on Vero cells. Briefly, eye swabs were collected by anaesthetizing mice and gently proptosing each eye and wiping a sterile cotton swab three times around the eye in a circular motion and twice over the centre of the cornea in an ‘X’ pattern. The swabs were place in 1 ml of DMEM containing 10% FBS, 1% penicillin/streptomycin and stored at −80 °C until being titred. Before titering, the swabs were thawed and vortexed for 30 s at maximum speed. Heparin (H3393) was purchased from Sigma-Aldrich and 5 μl of 25 μg μl −1 was applied directly to mouse eyes as a HPSE inhibitor when applicable. Clinical scoring of epithelial keratitis Seven days post ocular infection, the same observer applied fluorescein dye strips to the sclera of mouse eyes, examined corneas with a handheld slit-lamp biomicroscope and scored the severity of epithelial lesions according to the following established criteria [18] : 0, no epithelial lesion or punctate epithelial erosion; 1, stellate keratitis or residue of dendritic keratitis; 2, dendritic keratitis occupying less than one quarter of the cornea; 3, dendritic keratitis occupying one quarter to one half of the cornea; 4, dendritic keratitis extending over more than one half of the cornea. Human corneas Human donor corneoscleral buttons were obtained from the Illinois Eye Bank, Chicago, IL. The corneas were cultured and infected with 10 4 p.f.u. HSV-1 as previously described [65] with some modifications. Briefly, corneoscleral buttons were placed in a dish with medium, and virus diluted in 10 μl of medium was added to the corneal apex. Virus-containing media did not mix with the media in the dish. Corneal epithelial cells were harvested and lysed by scraping into 200 μl RIPA buffer with a scalpel blade. To minimize variability, eyes of the same donor were used as controls. Statistics Error bars of all figures represent s.e.m. of three independent experiments ( n =3), unless otherwise specified. Asterisks denote a significant difference as determined by Student’s t- test; * P <0.05, ** P <0.01, *** P <0.001, **** P <0.0001, ns, not significant. How to cite this article: Hadigal, S.R. et al. Heparanase is a host enzyme required for herpes simplex virus-1 release from cells. Nat. Commun. 6:6985 doi: 10.1038/ncomms7985 (2015).